A new clade of Asian Late Cretaceous long-snouted tyrannosaurids The iconic tyrannosaurids were top predators in Asia and North America during the latest Cretaceous, and most species had deep skulls that allowed them to generate extreme bite forces. Two unusual specimens of Alioramus from Mongolia seem to indicate a divergent long-snouted body plan among some derived tyrannosaurids, but the rarity and juvenile nature of these fossils leaves many questions unanswered. Here, we describe a remarkable new species of long-snouted tyrannosaurid from the Maastrichtian of southeastern China, Qianzhousaurus sinensis . Phylogenetic analysis places Qianzhousaurus with both species of Alioramus in a novel longirostrine clade, which was geographically widespread across latest Cretaceous Asia and formed an important component of terrestrial ecosystems during this time. The new specimen is approximately twice the size as both Alioramus individuals, showing that the long-snouted morphology was not a transient juvenile condition of deep-snouted species, but a characteristic of a major tyrannosaurid subgroup. Tyrannosauroids are among the most iconic animals in the fossil record. This group of large-bodied carnivorous dinosaurs, which includes Tyrannosaurus rex and its closest relatives, were the apex predators in Asia and North America during the final 20 million years of the Cretaceous, and were at the top of the food chain in these regions when a bolide impact (and perhaps other environmental changes) suddenly ended the age of non-avian dinosaurs 66 million years ago [1] , [2] , [3] . The vast majority of derived tyrannosauroids (tyrannosaurids) are characterized by deep skulls, thick teeth and large jaw muscles, features which allowed these dinosaurs to employ bite forces strong enough to crunch through the bones of even large-bodied prey species [4] , [5] , [6] , [7] . This unusual body plan is thought to have been the key to tyrannosaurid success [8] . A few enigmatic specimens from the Late Cretaceous (Maastrichtian) of Asia, however, suggest that a very different type of tyrannosaurid may have coexisted with these muscular, deep-skulled species during the final few million years of dinosaur evolutionary history. The holotypes of Alioramus remotus [9] and Alioramus altai [10] , [11] from Mongolia are both gracile animals with extremely long skulls relative to body size, with elongated snouts and thin teeth. It has been suggested recently that these fossils may represent a peculiar body plan among a handful of derived tyrannosaurids, indicative of different feeding styles and a lower position in the food chain relative to their coexisting deep-skulled cousins [10] , [11] . There is concern, however, because only two specimens of these long-snouted tyrannosaurids have been recovered, and both are juveniles, leading some workers to worry that they may represent transient longirostrine growth stages during the ontogeny of deeper-skulled species [12] . The extreme rarity of these animals, and their restriction to a narrow time interval in Mongolia, makes it difficult to test these hypotheses. We report the discovery of an aberrant new tyrannosaurid from the Late Cretaceous of southeastern China that is known from a remarkably complete and well-preserved skull, along with much of the vertebral column and appendicular skeleton. Other dinosaurs from the same horizon include the somphospondylan sauropod Gannansaurus sinesis [13] and several oviraptorosaurian theropods ( Banji long [14] ; Ganzhousaurus nankangensis [15] ; Jiangxisaurus ganzhouensis [16] ; Nankangia jiangxiensis [17] ). The new tyrannosaurid was the top predator in this terrestrial ecosystem. This tyrannosaurid possesses the characteristic long and low snout of both species of Alioramus , along with other features uniquely shared by these longirostrine taxa relative to deep-skulled tyrannosaurids. As a result, the three species are grouped together in their own distinct long-snouted clade by a phylogenetic analysis. The new species is larger (twice the body mass) and more skeletally mature than either specimen of Alioramus , which demonstrates that a long-snouted morphology was present in larger individuals and not likely to be a transient juvenile feature. The discovery of this species in southern China also shows that the long-snouted carnivores were geographically widespread across Asia during the latest Cretaceous, and formed an important (but hitherto overlooked) component of terrestrial ecosystems during this time. Systematic palaeontology Dinosauria Owen 1842 Theropoda Marsh 1881 Tetanurae Gauthier 1986 Coelurosauria von Huene 1914 Tyrannosauroidea Osborn, 1905 Alioramini Olskevsky, 1995, clade nov. Definition. The most inclusive clade containing A . remotus [9] , but not Tyrannosaurus rex [18] , Albertosaurus sarcophagus [18] or Proceratosaurus bradleyi [19] . Olshevsky [20] used the name Alioramini to refer to a monotypic tribe-level Linnean taxon for A . remotus , but we first use this name to refer to a novel clade of long-snouted tyrannosauroids. Diagnosis. Alioramini differs from all other tyrannosauroids in possessing an extremely long and low skull, in which the snout comprises 2/3 or more of the total skull length; an anteroposteriorly elongate maxillary fenestra (ratio of maximum anteroposterior length to maximum dorsoventral depth greater than 1.9); a series of pronounced, discrete rugosities on the nasal; 18 or more dentary teeth. Full synapomorphy is listed in Supplementary Note 3 . Included species. A . altai [10] , A . remotus [9] , Qianzhousaurus sinensis gen. et sp. nov. Qianzhousaurus sinensis gen . et sp. nov. Etymology. From Qianzhou, an ancient name of Ganzhou, where the fossils were discovered. Sin (Greek) China, refers to the specimen found from China. Holotype. A nearly complete skull and most of the left lower jaw (GM F10004-1); nine cervical vertebrae (GM F10004-2); three anterior dorsal vertebrae (GM F10004-3); 18 middle posterior caudal vertebrae (GM F10004-4); a complete right scapulocoracoid (GM F10004-5); part of the left scapulocoracoid (GM F10004-6); both partial ilia, a left femur and left tibia, a left partial fibula, a left astragalus and calcaneum and left metatarsals (GM F10004-7, 8). The specimens, which were found associated and represent a single individual, are housed at the Ganzhou Museum, Ganzhou City, Jiangxi Province, China. Measurements are provided in Supplementary Tables 1-5 . Locality and horizon. Nanxiong Formation (Upper Cretaceous, Maastrichtian) of Longling Town, Nankang, Ganzhou City, Jiangxi Province, China [21] . Diagnosis. Long-snouted tyrannosaurid tyrannosauroid with the following autapomorphies: large, discrete, window-like pneumatic fenestra on the ascending ramus of the maxilla; extremely reduced premaxilla (maximum anteroposterior length of the main body of the bone is ~2.2% of the total basal skull length, whereas other tyrannosaurids have measures of ~4.3–4.6%); absence of a pronounced vertical ridge on the lateral surface of the ilium (possibly shared with Raptorex kriegsteini [8] ). Comparative description The skull of Qianzhousaurus is well preserved and nearly complete, missing only a small portion of the orbital region on the right side ( Fig. 1 ). It is exceptionally long and low compared with other large-bodied tyrannosauroids like Tyrannosaurus and Albertosaurus [12] , [22] , [23] , but very similar in proportions to the longirostrine skulls of both species of Alioramus [9] , [10] , [11] . As in Alioramus , the preorbital (snout) region of the skull is elongated such that it is ~70% of the length of the entire skull ( Fig. 1 ), whereas this is ~60% in other large tyrannosaurids. Also as in Alioramus , the individual bones of the snout such as the maxilla and nasal (but not premaxilla) are elongated, whereas those of the posterior skull are of similar proportions to other large tyrannosaurids. The skull of Qianzhousaurus is 90 cm long anteroposteriorly when measured between the anterior edge of the premaxilla and the posteroventral corner of the quadrate in lateral view, compared with ~63 cm in the holotype of A . altai and a similar reconstructed measurement for the type of A . remotus [10] . 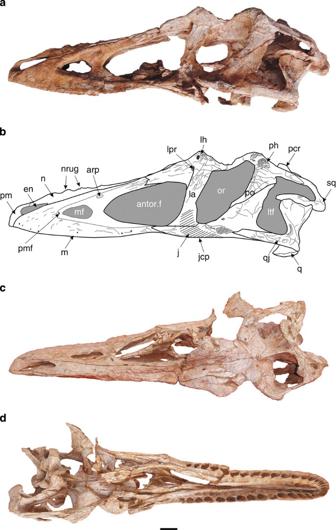Figure 1: Holotype skull ofQianzhousaurus sinensisgen. et sp. nov. (GM F10004-1). (a) Photograph in left lateral view, (b) line drawing in left lateral view, (c) photograph in dorsal view, (d) photograph in ventral view. antor.f, antorbital fenestra; arp, window-like pneumatic recess on the ascending ramus of the maxilla (autapomorphy); en, external naris; j, jugal; jcp, jugal cornual process; la, lacrimal; lh, lacrimal horn (cornual process); lpr, lacrimal pneumatic recess; ltf, lateral temporal fenestra; m, maxilla; mf, maxillary fenestra; n, nasal; nrug, nasal rugosities; or, orbit; pcr, parietal sagittal crest; ph, postorbital horn (cornual process); pmf, promaxillary fenestra; po, postorbital; q, quadrate; qj, quadratojugal; sq, squamosal. Scale bar, 5 cm. Figure 1: Holotype skull of Qianzhousaurus sinensis gen. et sp. nov. (GM F10004-1). ( a ) Photograph in left lateral view, ( b ) line drawing in left lateral view, ( c ) photograph in dorsal view, ( d ) photograph in ventral view. antor.f, antorbital fenestra; arp, window-like pneumatic recess on the ascending ramus of the maxilla (autapomorphy); en, external naris; j, jugal; jcp, jugal cornual process; la, lacrimal; lh, lacrimal horn (cornual process); lpr, lacrimal pneumatic recess; ltf, lateral temporal fenestra; m, maxilla; mf, maxillary fenestra; n, nasal; nrug, nasal rugosities; or, orbit; pcr, parietal sagittal crest; ph, postorbital horn (cornual process); pmf, promaxillary fenestra; po, postorbital; q, quadrate; qj, quadratojugal; sq, squamosal. Scale bar, 5 cm. Full size image The premaxilla is extremely reduced in size. Tyrannosauroids generally possess small premaxillae that are less than 10% of the total anteroposterior length of the maxilla (and at most 4–5% of the total anteroposterior length of the skull) [12] , [21] , [22] , [23] , [25] . Qianzhousaurus takes this reduction to the extreme, as its premaxilla is merely 2.2% of the basal length of the skull. Such size reduction is unexpected, given that the other bones of the snout are proportionally elongate in Qianzhousaurus compared with other tyrannosaurids (see above). The premaxilla houses four tooth sockets, which form a tooth row that is oriented mediolaterally such that all teeth are visible in anterior view, as is characteristic of tyrannosaurids [2] , [26] . The maxilla is extensively pneumatic. The maxillary fenestra is remarkably anteroposteriorly elongate, such that the ratio of its length to maximum depth is greater than 1.9 ( Fig. 1b ). This feature was previously held to be an autapomorphy of A . altai [10] , [11] , but its presence in Qianzhousaurus shows that it is a more widespread feature among long-snouted tyrannosaurids. Qianzhousaurus lacks the small accessory fenestra posterodorsal to the promaxillary fenestra that is autapomorphic of A . altai [10] , [11] . One of the most conspicuous features of the skull of Qianzhousaurus is the autapomorphic presence of an elongate, ovoid, window-like accessory pneumatic opening that pierces the lateral surface of the ascending ramus of the maxilla, posterodorsal to the maxillary fenestra and separated from the antorbital fenestra by a few centimeters ( Fig. 2b ). This may be related to a shallow depression on the ascending ramus of A . altai , held to be autapomorphic for that species, but comparatively the pneumatic fenestra in Qianzhousaurus is larger, located further posteriorly, oriented nearly vertically instead of horizontally, and a much more discrete opening with well-developed margins. The maxilla ( Fig. 1d ) has 15 alveoli, which are incrassate in shape (labiolingual width 60% or greater than the mesiodistal length) like those of large tyrannosaurids like Albertosaurus and Daspletosaurus , and unlike the thin ziphodont teeth of A . altai [2] . 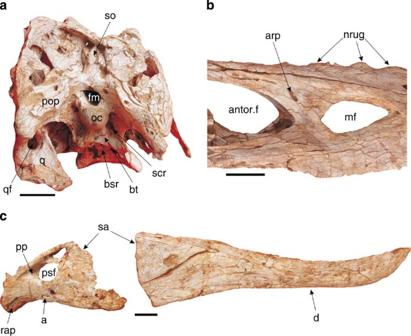Figure 2: Holotype skull ofQianzhousaurus sinensisgen. et sp. nov. (GM F10004-1). (a) Photograph of braincase in posterior view, (b) photograph of closeup of antorbital region of skull in right lateral view illustrating an autapomorphy of the species (arp) and a synapomorphy of Alioramini (nrug), (c) photograph of mandible in right lateral view. a, angular; antor.f, antorbital fenestra; arp, window-like pneumatic recess on the ascending ramus of the maxilla (autapomorphy); bsr, basisphenoid recess; bt, basal tubera; d, dentary; fm, foramen magnum; mf, maxillary fenestra; nrug, nasal rugosities; oc, occipital condyle; pop, paroccipital process; pp, pneumatic pocket; psf, posterior surangular foramen; q, quadrate; qf, quadrate foramen; rap, retroarticular process; sa, surangular; scr, subcondylar recess; so, supraoccipital. Scale bar, 5 cm. Figure 2: Holotype skull of Qianzhousaurus sinensis gen. et sp. nov. (GM F10004-1). ( a ) Photograph of braincase in posterior view, ( b ) photograph of closeup of antorbital region of skull in right lateral view illustrating an autapomorphy of the species (arp) and a synapomorphy of Alioramini (nrug), ( c ) photograph of mandible in right lateral view. a, angular; antor.f, antorbital fenestra; arp, window-like pneumatic recess on the ascending ramus of the maxilla (autapomorphy); bsr, basisphenoid recess; bt, basal tubera; d, dentary; fm, foramen magnum; mf, maxillary fenestra; nrug, nasal rugosities; oc, occipital condyle; pop, paroccipital process; pp, pneumatic pocket; psf, posterior surangular foramen; q, quadrate; qf, quadrate foramen; rap, retroarticular process; sa, surangular; scr, subcondylar recess; so, supraoccipital. Scale bar, 5 cm. Full size image The nasals are fused ( Fig. 1a,c ) and vaulted as in all tyrannosaurids, and they share a striking feature with both species of Alioramus : a series of pronounced, rugose mounds along the midline of the dorsal surface. The cornual process of the lacrimal is a discrete projection that extends above the skull roof as in most other tyrannosaurids, whereas it is autapomorphically expressed as a small, conical ‘horn’ in A . altai [11] and absent in Tarbosaurus and Tyrannosaurus [2] , [22] , [23] , [26] . The jugal bears a subtle ventrally-projecting cornual process along its ventral margin but lacks the laterally-projecting horn that is autapomorphic of A . altai [10] , [11] . The cornual process of the postorbital is a large swelling that extends past the dorsal margin of the bone to project above the skull roof, similar to the condition in other tyrannosaurids but unlike the smaller processes of both species of Alioramus , which are limited to a slight rugose rim at the posterodorsal corner of the orbit [2] , [8] . The ventral ramus of the postorbital does not markedly protrude into the orbit as a suborbital flange (although an incipient version of the flange is present), an ontogenetically controlled character that is seen in adults of large tyrannosaurids like Tyrannosaurus but absent (or incipient) in juveniles and subadults, including the holotype of A . altai [2] , [27] . There is a large pneumatic recess on the ventral surface of the squamosal, as in tyrannosaurids generally, and a funnel-like foramen on the anterior surface of the quadrate immediately above the condyles that leads into an internal recess, as in most tyrannosauroids [28] . The rectangular frontals are wider than long and sport a small nasal process anteriorly, as in most tyrannosaurines but not albertosaurines and non-tyrannosaurids [2] , [8] . Unlike the tyrannosaurines Daspletosaurus , Tarbosaurus and Tyrannosaurus , however, the frontal does contribute to the orbital rim [2] , [8] , [27] . The occipital surface of the braincase faces strongly posteroventrally as in other tyrannosaurids [8] . The supraoccipital is not bifurcated dorsally as it is in many large tyrannosaurids [23] , [27] , but does make a small contribution to the dorsal rim of the foramen magnum, as is normal for tyrannosauroids [2] . The fossa for cranial nerves X–XII on the exoccipital–opisthotic is deep and funnel-like. The basal tubera are dorsoventrally deeper than the occipital condyle ( Fig. 2a ), as is normal for tyrannosaurids, and are penetrated by several foramina that lead into the subcondylar recess, as is seen in most tyrannosaurids but not Tarbosaurus and Tyrannosaurus [2] , [22] , [23] , [26] . The basisphenoid recess is partially visible in posterior view, not compressed anteroposteriorly and widely visible in posterior view as in Tarbosaurus , Tyrannosaurus and Teratophoneus [2] , [22] , [23] . The long, gracile dentary ( Fig. 2c ) is unexpanded anteriorly and lacks the projecting ‘chin’ at its anteroventral margin, a feature that is present in all other tyrannosaurids [2] . It contains 18 alveoli, an identical count to the holotype of A . remotus [9] but fewer than the 20 tooth positions in the holotype of A . altai [10] , [11] . Tyrannosaurus rex possesses 12–17 dentary teeth depending on ontogeny, and to our knowledge no other tyrannosauroid specimens exhibit more than 17 dentary teeth [22] , [27] , [29] , [30] . The posterior surangular foramen is enormous as in tyrannosaurids and proximal outgroups, and is bordered posterodorsally by a deep pneumatic pocket like that present in A . altai and many other tyrannosaurids [28] . The retroarticular process of the articular is short and there is no smooth non-articular region between the glenoid and jaw depressor muscle attachment site, both of which are characteristic of most tyrannosauroids [31] . The cervical vertebrae are highly pneumatic ( Fig. 3a ). There are several pneumatic foramina and fossae on the anterior surface of the axial neural spine, which are absent in A . altai but present in all other tyrannosaurines [2] . All preserved dorsal vertebral centra bear pneumatic foramina and are anteroposteirorly longer than tall dorsoventrally, which is the case in most tyrannosauroids but distinct from the proportionally tall centra of Daspletosaurus , Tarbosaurus and Tyrannosaurus [2] , [26] . None of the caudals exhibit pneumatic foramina or other indicators of pneumaticity ( Fig. 3b ), and the neural spine bases of the anterior caudals are level with or posterior to the posterior edge of the centrum, which is also the case in other tyrannosaurines [2] . 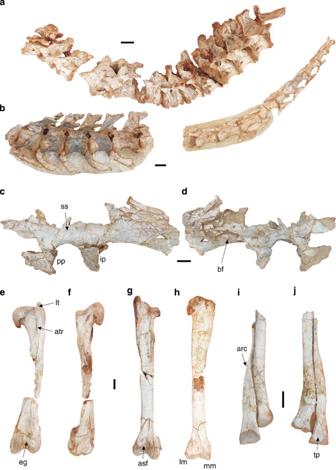Figure 3: Holotype postcranium ofQianzhousaurus sinensisgen. et sp. nov. (F10004-2~GM F10004-8). (a) Photographs of cervical and dorsal vertebrae in left lateral view, (b) photographs of middle-to-posterior caudal vertebrae in left lateral view, (c) photograph of left ilium in lateral view, (d) photograph of left ilium in medial view, (e) photograph of left femur in anterior view, (f) photograph of left femur in medial view, (g) photograph of left tibia in anterior view, (h) photograph of left tibia in posterior view, (i) photograph of left metatarsus in extensor (anterior) view, (j) photograph of left metatarsus in flexor (posterior) view. arc, arctometatarsalian condition of metatarsal III; asf, fossa on anterior surface of astragalus; atr, accessory trochanter; bf, brevis fossa; eg, extensor groove; ip, ischial peduncle; lm, lateral malleolus; mm, medial malleolus; pp, pubic peduncle, ss, smooth lateral surface of ilium; tp, triangular platform on flexor surface of metatarsal III. Scale bar, 5 cm. Figure 3: Holotype postcranium of Qianzhousaurus sinensis gen. et sp. nov. (F10004-2~GM F10004-8). ( a ) Photographs of cervical and dorsal vertebrae in left lateral view, ( b ) photographs of middle-to-posterior caudal vertebrae in left lateral view, ( c ) photograph of left ilium in lateral view, ( d ) photograph of left ilium in medial view, ( e ) photograph of left femur in anterior view, ( f ) photograph of left femur in medial view, ( g ) photograph of left tibia in anterior view, ( h ) photograph of left tibia in posterior view, ( i ) photograph of left metatarsus in extensor (anterior) view, ( j ) photograph of left metatarsus in flexor (posterior) view. arc, arctometatarsalian condition of metatarsal III; asf, fossa on anterior surface of astragalus; atr, accessory trochanter; bf, brevis fossa; eg, extensor groove; ip, ischial peduncle; lm, lateral malleolus; mm, medial malleolus; pp, pubic peduncle, ss, smooth lateral surface of ilium; tp, triangular platform on flexor surface of metatarsal III. Scale bar, 5 cm. Full size image The scapula and coracoid are fused, and the scapula has an elongate, strap-like blade whose length is more than 10 times its minimal depth, as in other tyrannosaurids [8] . The ilium has an enormous antitrochanter ( Fig. 3c,d ), a squared-off postacetabular process, and pubic and ischial peduncles with nearly identical anteroposteror lengths at their bases, all of which are common in tyrannosaurids [2] . Unlike nearly all other tyrannosauroid specimens, however, the lateral surface of the iliac blade lacks a prominent vertical crest above the acetabulum. To our knowledge, the only other tyrannosauroid specimen to lack this crest is the holotype of Raptorex kriegsteini , which is a small juvenile individual [8] . The femur ( Fig. 3e,f ) is approximately 70 cm long, larger than the 56-cm-long femur of the A . altai holotype [10] , [11] . The lesser trochanter extends to the same level proximally as the greater trochanter, the accessory trochanter on the anterior margin of the lesser trochanter is reduced to a subtle convexity, and the extensor groove distally is a deep U-shaped cleft in distal view. The lateral malleolus of the tibia extends to the same level distally as the medial malleolus ( Fig. 3g,h ), which is also the case in A . altai but unlike the much more extensive lateral malleoli of other tyrannosaurids [2] . The pes is arctometatarsalian ( Fig. 3i,j ), and metatarsal III has a convex expansion along the medial surface of the shaft and a raised subtriangular platform proximal to the condyles on the flexor surface of the bone, all of which are characteristic of tyrannosaurids but not more basal tyrannosauroids like Dilong , Eotyrannus and Guanlong [2] , [8] . Maturity of the specimen Unfortunately, a histological age estimate for the Qianzhousaurus type is not available at this time, because of concerns about destructive sampling of the specimen. However, the holotype of Qianzhousaurus is demonstrably larger and more mature than the holotypes of both species of Alioramus . The femur of the Qianzhousaurus type is approximately 70 cm long, 25% larger than the 56-cm-long femur of the A . altai type. On the basis of equations that predict body mass from femur length [32] , the holotype individual of Qianzhousaurus had approximately twice the body mass as the holotype individual of A . altai (757 versus 369 kg). Furthermore, the skull of the Qianzhousaurus type is approximately 43% longer than the A . altai type, which is nearly identical in size (within 3–5%) of the reconstructed skull length of the A . remotus type. Several lines of evidence indicate that the type individual of Qianzhousaurus was more skeletally mature than either Alioramus specimen (see Supplementary Fig. 1 and Supplementary Note 2 for a detailed discussion). It exhibits a greater degree of fusion of the skull roof bones (nasals) and braincase, and for some sutures that are known to close during tyrannosaurid ontogeny it exhibits a closed condition whereas the sutures are open in the Alioramus specimens. It also possesses the more mature version of numerous discrete characters that are known to change during the ontogeny of tyrannosaurids and close outgroups [26] , [27] , [30] . These include: a large and swollen lacrimal cornual process (not the small conical ‘hornlet’ of A . altai ), a bulbous postorbital cornual process that extends past the dorsal edge of the skull roof (compared with the subtle ridge-like processes immediately posterodorsal to the orbit in both species of Alioramus , characteristic of juvenile tyrannosaurids), thickened incrassate teeth (compared with the thin ziphodont teeth of the Alioramus specimens and other juveniles) and fewer teeth in the maxilla (15 versus 16 for A . remotus and 17 for A . altai ) and dentary (18, the same as in A . remotus but versus 20 in A . altai ). Although the long-snouted body plan of alioramins deviates from the bauplan of other large-bodied tyrannosauroids, they most likely experienced a similar sequence of ontogenetic changes as their deep-snouted relatives. The aforementioned patterns of discrete character change during tyrannosauroid ontogeny are seen in a range of tyrannosaurids and close non-tyrannosaurid outgroups of different body sizes, ages and geographic localities ( Bistahieversor , Gorgosaurus , Tyrannosaurus ) [26] , [27] , [30] , indicating that this pattern is a conservative plesiomorphic condition for Tyrannosauridae and close outgroups. Furthermore, Brusatte et al . [10] demonstrated that A . altai underwent a similar sequence of discrete ontogenetic changes as Tyrannosaurus , based on a quantitative ontogenetic cladistic analysis that placed the 9-year-old A . altai type (aged by histology) intermediate between Tyrannosaurus individuals younger and older than 9 years old (also aged by histology). In other words, A . altai had a set of ontogenetically variable features expected for a ca. 9-year-old Tyrannosaurus . When the type of Qianzhousaurus is added to this analysis (see Supplementary Note 2 ), it groups with subadult and adult Tyrannosaurus in a more derived (mature) position on the tree than the A . altai type. This is quantitative support that the holotype of Qianzhousaurus is more mature than that of A . altai , assuming that the Tyrannosaurus ontogeny sequence is applicable to alioramins as argued above. Although the type of Qianzhousaurus is more mature than both Alioramus specimens, it still does not appear to be fully grown, as the neurocentral sutures between the cervical and dorsal vertebrae are only partially fused. It is possible that the Qianzhousaurus type is a more mature member of either A . altai or A . remotus , but because it possesses traits (here considered autapomorphies) not seen in the holotypes of these species, lacks traits (autapomorphies) of the Alioramus species and was found at a geographically disparate locality, we recognize it as a diagnostic taxon. Future discoveries, however, will better test this hypothesis. The long-snouted body plan We conducted a linear regression of skull length versus femur length in tyrannosaurids, in order to gauge whether the holotypes of Qianzhousaurus sinensis and A . altai have a longer skull relative to femur length (a body size proxy) than other tyrannosaurids, which would be evidence for a distinctive longirostrine bauplan (see Supplementary Note 1 ). This is the first statistical analysis testing the uniqueness of the long-snouted body plan. The analysis recovers a highly significant relationship between skull length and femur length ( r =0.95944, P <0.0001) and places the types of Qianzhousaurus sinensis and A . altai outside of the 95% confidence intervals of the best fit line, quantitatively demonstrating that these specimens have significantly longer skulls relative to their femur lengths than non-long-snouted tyrannosaurids ( Fig. 4 ). The Qianzhousaurus type has a skull that is 35% longer than a Tarbosaurus bataar specimen of identical femur length, providing further evidence of the novelty of the long-snouted bauplan and the conclusion that Qianzhousaurus is not a juvenile Tarbosaurus . 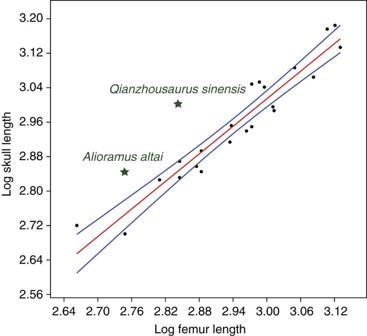Figure 4: Linear regression of the logarithms of skull length versus femur length for several tyrannosaurid specimens. There is a highly significant relationship between skull and femur lengths (24 specimens,r=0.95944,P<0.0001). The two alioramin specimens are denoted by stars. Note that the holotypes ofQianzhousaurusandA.altaifall above the regression line and outside of the 95% confidence intervals, meaning that they have longer skulls relative to their skull lengths than other tyrannosaurids. Note also thatQianzhousaurushas a longer skull length than two specimens of other tyrannosaurids that have nearly exactly the same femur length andA.altaihas a longer skull length than a tyrannosaurid specimen of nearly identical femur length. Figure 4: Linear regression of the logarithms of skull length versus femur length for several tyrannosaurid specimens. There is a highly significant relationship between skull and femur lengths (24 specimens, r =0.95944, P <0.0001). The two alioramin specimens are denoted by stars. Note that the holotypes of Qianzhousaurus and A . altai fall above the regression line and outside of the 95% confidence intervals, meaning that they have longer skulls relative to their skull lengths than other tyrannosaurids. Note also that Qianzhousaurus has a longer skull length than two specimens of other tyrannosaurids that have nearly exactly the same femur length and A . altai has a longer skull length than a tyrannosaurid specimen of nearly identical femur length. Full size image Phylogenetic analysis We added Qianzhousaurus sinensis to the phylogenetic analysis of Brusatte and Benson [33] , a modified version of the analysis of Brusatte et al . [2] The analysis includes a broad sample of 21 tyrannosauroids scored for 317 morphological characters ( Supplementary Data 2 ). A parsimony analysis resulted in two most parsimonious trees (586 steps, consistency index=0.628, retention index=0.834). The strict consensus tree ( Fig. 5 ) places Qianzhousaurus sinensis , A . altai and A . remotus in a subclade of long-snouted tyrannosaurids at the base of Tyrannosaurinae, sister taxon to the clade of Teratophoneus , Daspletosaurus , Tarbosaurus and Tyrannosaurus . The long-snouted clade, which is here termed Alioramini, is strongly supported (jackknife percentage=87%, Bremer support=4) and united by several synapomorphies, including discrete rugosities on the nasal and 18 or more dentary teeth (see full list in Supplementary Note 3 ). The three alioramin taxa comprise a polytomy in the strict consensus, because one most parsimonious tree places Qianzhousaurus as the sister taxon to an A . altai + A . remotus clade, whereas the other places Qianzhousaurus and A . altai in a clade exclusive of A . remotus . This uncertainty is almost certainly due to large amounts of missing data in A . remotus , a taxon known only from a fragmentary holotype that has never been fully described in the literature. 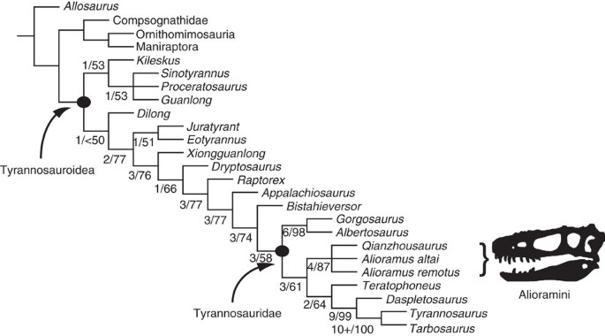Figure 5: Phylogenetic relationships of long-snouted tyrannosauroids. Strict consensus of the two most parsimonious trees. Trees recovered from the primary phylogenetic analysis (586 steps, consistency index=0.628, retention index=0.834). Numbers next to nodes denote Bremer supports and jackknife values (absolute frequencies, 36% character removal probability, 1,000 replicates). The novel clade of long-snouted tyrannosauroids, Alioramini, is indicated. Figure 5: Phylogenetic relationships of long-snouted tyrannosauroids. Strict consensus of the two most parsimonious trees. Trees recovered from the primary phylogenetic analysis (586 steps, consistency index=0.628, retention index=0.834). Numbers next to nodes denote Bremer supports and jackknife values (absolute frequencies, 36% character removal probability, 1,000 replicates). The novel clade of long-snouted tyrannosauroids, Alioramini, is indicated. Full size image As a supplementary analysis to assess the robustness of our phylogenetic results, we also added Qianzhousaurus to an alternative tyrannosauroid phylogenetic analysis presented by Loewen et al . [3] (see Supplementary Note 3 and Supplementary Data 3 ). Agreeing with our primary analysis, this procedure also recovered Qianzhousaurus , A . altai and A . remotus in a subclade of long-snouted taxa, with a minor difference that this clade is placed immediately outside of Albertosaurinae+Tyrannosaurinae rather than as basal tyrannosaurines. This provides additional support for our primary phylogenetic conclusion: that Qianzhousaurus is a part of a restricted subgroup of long-snouted tyrant dinosaurs. The discovery of Qianzhousaurus helps clarify the anatomy and systematics of the long-snouted tyrannosaurids, some of the rarest and most poorly understood large-bodied theropods in the fossil record. Qianzhousaurus is only the third specimen of a longirostrine tyrannosaurid from the Late Cretaceous of Asia, and our phylogenetic analysis indicates that this and the other two specimens (the holotypes of A . altai and A . remotus ) form a clade of long-snouted predators at the base of Tyrannosaurinae, the tyrannosaurid subclade that also includes Tyrannosaurus and Tarbosaurus . Although close relatives of the iconic Tyrannosaurus , these longirostrine species represent a distinct experiment in tyrannosaurid evolution. Their long and slender snouts, heavily ornamented skulls, and gracile skeletons constitute a unique body plan differing from the more robustly constructed, deep-skulled bauplan characteristic of most other tyrannosaurids, held to be integral to their role as apex predators and their evolutionary success [8] . The long-snouted body plan was not a marginal evolutionary outlier restricted to one or two Late Cretaceous species, but characteristic of an entire subclade of tyrannosaurids whose membership is growing as new fossil evidence from Asia continues to accumulate. Not only were longirostrine tyrannosaurids more taxonomically diverse than previously thought, they were also more geographically widespread, and appear to have formed an important component of Asian terrestrial ecosystems during the latest Cretaceous. Previous discoveries of Alioramus are known exclusively from the Maastrichtian Nemegt Formation (or apparently equivalent beds) of Mongolia [9] , [10] , [11] . Qianzhousaurus was discovered in similar-aged rocks approximately 3,000 km southeast of the classic Nemegt localities, in the Jiangxi Province of China. Although long-snouted alioramin tyrannosaurids are still incredibly rare in the fossil record, their discovery at widely disparate sites across Asia suggests that they were a broadly distributed group and a standard component of dinosaurian ecosystems in Asia during the few million years before the end of the Cretaceous. Alioramins coexisted across Asia with Tarbosaurus (and potentially other species of more traditional, deep-snouted tyrannosaurids [34] ), and their divergent body plans may have allowed them to partition niches. Interestingly, all known specimens of long-snouted alioramins have pronounced rugosities on the nasals, which are a synapomorphy uniting the clade. This distinctive form of ornamentation is present in both smaller-bodied (and presumably ontogenetically younger) specimens like the holotypes of A . remotus and A . altai , and much larger and more mature specimens like the holotype of Qianzhousaurus . Tyrannosauroids generally possess a variety of cranial ornaments, with distinct horns, bosses or rugosities regularly occurring on the lacrimal, postorbital and jugal, suggesting that they were highly visual animals that relied on these structures for display and communication. Because the unique nasal bosses of alioramins are present at multiple ontogenetic stages, including immature subadults, it is possible that they may have been signals to distinguish these animals from other coexisting large-bodied tyrannosaurids [35] , [36] . Alternatively, they may have been an idiosyncratic sexual display structure limited to this one tyrannosaurid subgroup. Although alioramins seem to have been diverse and widespread in latest Cretaceous Asia, there is no strong evidence that similar longirostrine tyrannosaurids were present in North America during this time. The controversial taxon ‘ Nanotyrannus ’, held to be either a distinct species of small-bodied long-snouted tyrannosaurid [37] or a juvenile Tyrannosaurus rex [27] , [30] , is potentially one such animal. However, ‘ Nanotyrannus ’ does not exhibit the extreme longirostrine morphology of alioramins. Its snout is approximately 65% of total skull length, compared with ~70% in alioramins, and its skull is proportionally taller than in alioramins (depth at posterior margin of antorbital fenestra divided by total skull length is ~30%, compared with ~25% in alioramins) [27] , [37] . In addition, ‘ Nanotyrannus ’ lacks three synapomorphies of Alioramini: discrete nasal rugosities, an enlarged maxillary fenestra and 18 or more dentary teeth [27] , [33] , [38] . Therefore, if ‘ Nanotyrannus ’ is a distinct taxon, it does not appear to be a member of Alioramini, and may represent a separate acquisition of longirostrine morphology among tyrannosaurids. The apparent lack of long-snouted tyrannosaurids in the latest Cretaceous of North America provides further evidence that Asian and North American faunas at this time, although very similar in many respects, were noticeably distinct. Ceratopsids, which were widespread and diverse across western North America during the Campanian–Maastrichtian, are represented by only a single Asian specimen [39] . Conversely, sauropods were remarkably rare in the Maastrichtian of North America but more diverse in Asia [40] . North America and Asia clearly experienced faunal interchange during the latest Cretaceous, but the presence of the inland Western Interior Sea, extensive mountain building and potential biogeographic provincialism may have uniquely shaped North American dinosaur evolution relative to other regions of the northern hemisphere, and the world, at this time [41] . It appears as if Asian and North American dinosaurs were undergoing distinct biodiversity trajectories during the latest Cretaceous [42] , [43] , meaning that the well-sampled North American record, which has long been used as a standard to understand dinosaur evolution during the run-up to their extinction, may not be a reasonable proxy for the global record. The type of Qianzhousaurus is considerably larger ( ca. twice the body mass) and more mature than the holotypes of both species of Alioramus , thereby giving the first clear insight into the size and morphology of a larger-bodied, non-juvenile alioramin. There has been some concern that the holotypes of A . altai and A . remotus may represent juveniles of previously known tyrannosaurids (possibly the coeval Tarbosaurus ) rather than distinct taxa [44] , [45] . Both Alioramus specimens are juvenile individuals, as confirmed by bone histology in the case of the A . altai holotype [10] , and juvenile tyrannosaurids are known to have proportionally longer and shallower skulls, more gracile bones and more teeth than conspecific adults [27] , [30] . The discovery of Qianzhousaurus provides strong evidence that alioramins are distinct taxa with an unusual long-snouted bauplan resulting from evolutionary divergence, not ontogenetic growth. Although the Qianzhousaurus type is much larger and more mature than either specimen of Alioramus , it still possesses the characteristic long-snouted skull morphology. Furthermore, when the type individual of Qianzhousaurus is included in a regression of skull length versus femur length in tyrannosaurids [45] , it falls well above the regression line and outside the 95% confidence intervals as defined by other tyrannosaurids ( Fig. 4 ). In other words, Qianzhousaurus has a much longer skull than other tyrannosaurid individuals with similar femur lengths (a tyrannosaurine and albertosaurine in the analysis with nearly identical femur lengths have skulls that are 74.0 cm and 67.8 cm long between the premaxilla and distal end of the paroccipital process, respectively, compared with 100 cm in Qianzhousaurus ). This is also true of the type individual of A . altai , and indicates that during their growth trajectory alioramins consistently had skulls that were substantially longer than similarly-sized non-alioramin tyrannosaurids. In summary, the discovery of Qianzhousaurus demonstrates that long-snouted tyrannosaurids were a geographically widespread and taxonomically diverse component of Asian terrestrial ecosystems during the latest Cretaceous, with a statistically significant longirostrine body plan compared with more traditional deep-snouted tyrannosaurids that was not merely a transient juvenile feature. Previous examples of long-snouted tyrannosaurids were limited to two very young, small individuals from a small region of Mongolia [9] , [10] , [11] , but the Chinese Qianzhousaurus demonstrates that these aberrant tyrannosaurids ranged across Asia during the final few million years of the Age of Dinosaurs, retained their longirostrine morphology much later into maturity, and comprised a distinct tyrannosaurid subclade whose membership will probably continue to grow as the Asian dinosaur record becomes better sampled. Ontogenetic analysis To quantitatively compare the ontogenetic maturity stage of the type of Qianzhousaurus sinensis with the type of A . altai and other tyrannosaurids, we added the Qianzhousaurus specimen to a discrete character ontogenetic analysis presented by Brusatte et al . [10] , which is based on an earlier analysis [30] for Tyrannosaurus . This procedure was used previously to determine the maturity state of the A . altai holotype [10] . It gives a reasonable estimate of the Tyrannosaurus growth stage with which the Qianzhousaurus type corresponds to, and permits quantitative comparison of the relative ontogenetic stages of the Qianzhousaurus and A. altai types, based on the assumption that they follow a similar growth trajectory to Tyrannosaurus (which was argued to be the case by Brusatte et al . [10] ). The dataset includes 84 ontogenetically variable characters scored for seven ingroup taxa (the Qianzhousaurus and A. altai types and five specimens of Tyrannosaurus with known histological ages). The matrix was analysed in TNT v. 1.1 (ref. 46 ) under an exhaustive search. See Supplementary Figure 2 , Supplementary Note 2 , and Supplementary Data 1 for further details. Skull versus femur regression We added the types of Qianzhousaurus sinensis and A . altai to a dataset of skull and femur lengths for 22 other tyrannosaurid specimens (all specimens with skull and femur measurements that were available to us; Supplementary Table 6 ) [45] , [47] . We performed a linear regression analysis and calculated 95% confidence intervals in PAST v 2.17 (ref. 48 ). Phylogenetic analysis To specify the phylogenetic relationships of Qianzhousaurus sinensis , we included it in the phylogenetic data matrix of Brusatte and Benson [33] , an updated version of the dataset of Brusatte et al . [2] Three new characaters were added to encapsulate features of the maxilla, nasal and dentary that characterize long-snouted tyrannosaurids ( Supplementary Note 3 ). The dataset ( Supplementary Data 1 ) was run in TNT v. 1.1 (ref. 46 ), first using a ‘New Technology’ search (using sectorial search, ratchet, tree drift and tree fuse options with default parameters) to find a minimum length tree in 10 replicates, which aims to initially sample as many tree islands as possible. The resultant most parsimonious trees were then analysed under traditional TBR branch swapping, which more fully explores each tree island. Jackknife resampling (1,000 replicates, 36% character removal probability) and Bremer supports were used to assess clade support. A supplementary phylogenetic analysis was run in which Qianzhousaurus sinensis was added to the recent dataset of Loewen et al . [3] , which was analysed under the same protocols as the primary analysis (see Supplementary Fig. 3 , Supplementary Note 3 , Supplementary Data 3 ). Nomenclatural acts This published work and the nomenclatural acts it contains have been registered in ZooBank, the proposed online registration system for the International Code of Zoological Nomenclature (ICZN). The ZooBank LSID (Life Science Identifiers) can be resolved and the associated information viewed through any standard web browser by appending the LSID to the prefix ' http://zoobank.org/' . The LSID for this publication is: urn:lsid:zoobank.org:pub:D1FCC7C1-C3A2-41DB-B326-4EE87D1DC3AC. How to cite this article: Lü, J. et al . A new clade of Asian Late Cretaceous long-snouted tyrannosaurids. Nat. Commun. 5:3788 doi: 10.1038/ncomms4788 (2014).